Reconstructing plate-motion changes in the presence of finite-rotations noise Understanding lithospheric plate motions is of paramount importance to geodynamicists. Much effort is going into kinematic reconstructions featuring progressively finer temporal resolution. However, the challenge of precisely identifying ocean-floor magnetic lineations, and uncertainties in geomagnetic reversal timescales result in substantial finite-rotations noise. Unless some type of temporal smoothing is applied, the scenario arising at the native temporal resolution is puzzling, as plate motions vary erratically and significantly over short periods (<1 Myr). This undermines our ability to make geodynamic inferences, as the rates at which forces need to be built upon plates to explain these kinematics far exceed the most optimistic estimates. Here we show that the largest kinematic changes reconstructed across the Atlantic, Indian and South Pacific ridges arise from data noise. We overcome this limitation using a trans-dimensional hierarchical Bayesian framework. We find that plate-motion changes occur on timescales no shorter than a few million years, yielding simpler kinematic patterns and more plausible dynamics. Plate motions shape Earth's surface through time. Knowledge of these kinematics is therefore of paramount importance to make geodynamic inferences on sea-level change [1] , [2] , interactions between mantle plumes and the lithosphere [3] and dynamic topography [1] , [4] , [5] , [6] among others. Over the last decades great efforts have been made to reconstruct Earth's plate motions at progressively finer temporal resolution from observations of the ocean-floor spreading [7] . In particular, the kinematics of the Eurasia/North America (EU/NA), India/Somalia (IN/SO) and Pacific/Antarctica (PA/AN) spreading systems since mid-/late Cenozoic have been recently reconstructed at unprecedented temporal resolution [8] , [9] , [10] from finite rotations of Earth's ocean-floor. These map the imprints of past geomagnetic inversions, therefore providing the cumulative displacement between two adjacent spreading plates—in the form of total angle opened and average geographical position of the rotation axis from some time in the geological past, through to the present day. It is known, however, that these measurements feature substantial noise, which is the unknown finite-rotation fraction unrelated to actual plate motions. Noise arises mainly from the challenge of identifying precisely magnetic lineations of the ocean-floor, often from insufficiently long segments [11] of slowly spreading ridges, and partly from the calibration accuracy of geomagnetic reversal timescales [12] , [13] . In theory one would need a statistically significant number of repeated measurements of each finite rotation to minimise the associated noise. In practice this becomes unfeasible because finite rotations are derived from costly marine and airborne magnetic surveys. In the past, the issue of data noise might have been deemed of second-order importance, because finite rotations were typically reconstructed at resolutions of ∼ 10 Myr [14] . This yields small noise-to-signal ratios when computing Euler vectors directly by differentiation, with respect to time, of stage rotations obtained from two consecutive finite-rotation matrices. However, as finite rotations are reconstructed at progressively higher temporal resolution (<1 Myr) [8] , [9] , [10] , data noise becomes a major challenge to overcome. To date there is no solution to this problem, and the standard practise has been to smooth temporal series of single measurements [8] , [9] , [10] by averaging over 2 to 5 Myr-long time intervals, in the hope of isolating true plate motions and their temporal changes. Doing so, however, downgrades the native resolution of data-sets and, more importantly, does not provide unique kinematic reconstructions, because different averaging time-windows would yield different results. On the other hand, plate kinematics derived directly from finite rotations present an unexpected tectonic scenario, in that Euler vectors of relative motions vary erratically with no consistent trend over geologically short periods of <1 Myr ( Fig. 1a and Supplementary Figs S1a and S2a ). Consequently, spreading rates across the mid-Atlantic, Carlsberg and PA/AN ridges at the maximum resolution permitted by the data appear to change significantly through time ( Fig. 1b and Supplementary Figs S1b and S2b ), posing a limit to our ability of making geodynamic inferences from kinematic reconstructions. In fact, as plate motions readjust virtually instantaneously to temporal changes in the torque balance, the rates at which torques must vary to generate the observed changes in Euler vectors far exceed the most optimistic estimates, derived from simple geodynamic arguments ( Supplementary Information ), of those associated with the descent of slabs into the Earth's mantle [15] or the building of tectonic forces along plate margins [16] ( Fig. 1c and Supplementary Figs S1c and S2c ). 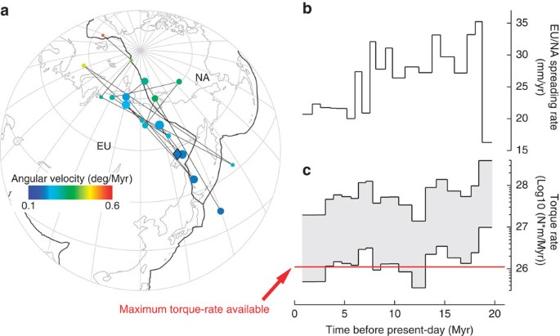Figure 1: Reconstructed plate kinematics and dynamic inferences. (a) Euler poles (dots) for the relative motion of the Eurasian plate (EU) with respect to fixed North America plate (NA) since∼20 Ma, reconstructed from finite rotations of the ocean-floor along the mid-Atlantic ridge. Euler poles are colour-coded according to their angular velocity. Symbol size increases from the oldest to the youngest (shown as diamond) Euler pole reconstructed. EU and NA plate margins are in black. Coastlines are in grey. (b) EU/NA spreading rate reconstructed at (28°W, 45°N), showing significant variations over geologically short periods. (c) Range of torque variation rates (grey area between black lines) required upon EU to explain the reconstructed Euler vector temporal changes. The largest Euler vector changes require torques variation rates significantly above reasonable estimates of the maximum available (red line). Figure 1: Reconstructed plate kinematics and dynamic inferences. ( a ) Euler poles (dots) for the relative motion of the Eurasian plate (EU) with respect to fixed North America plate (NA) since ∼ 20 Ma, reconstructed from finite rotations of the ocean-floor along the mid-Atlantic ridge. Euler poles are colour-coded according to their angular velocity. Symbol size increases from the oldest to the youngest (shown as diamond) Euler pole reconstructed. EU and NA plate margins are in black. Coastlines are in grey. ( b ) EU/NA spreading rate reconstructed at (28°W, 45°N), showing significant variations over geologically short periods. ( c ) Range of torque variation rates (grey area between black lines) required upon EU to explain the reconstructed Euler vector temporal changes. The largest Euler vector changes require torques variation rates significantly above reasonable estimates of the maximum available (red line). Full size image Here, we tackle noise in finite rotations by using a trans-dimensional hierarchical Bayesian framework [17] , [18] , [19] , [20] , [21] (Methods). We find that changes in the temporal trends of plate motions occur on timescales no shorter than a few million years, yielding simpler kinematic patterns and more plausible dynamics. Upon noise reduction, a spectral analysis of spreading-rate records since mid/late Cenozoic rules out kinematic changes over periods <0.5–1 Myr. This has important implications for the figure of contemporary plate motions observed from space geodesy [22] , [23] , [24] , which must have remained stable for longer than previously thought. Trans-dimensional hierarchical Bayesian formulation If relative plate motions remained stable over time, the rotation axis associated with finite-rotations temporal series would be fixed. Similarly, the total angle opened between plates would increase linearly, or alternatively the residual with respect to the linear trend imposed by the oldest finite rotation reconstructed would be null. Instead, if the angular velocity varied, or if the rotation axis wandered (or both) during the geological past, finite rotations will exhibit a departure of the residual angle from its linear trend, or a pronounced shift of the axis position (or both simultaneously). The inference framework used here allows us to isolate the fractions of residual angle and axis position likely related to plate-motion changes from those likely due to noise. We initially construct an ensemble [25] of millions of possible models describing the temporal evolution of finite-rotation residual angle, latitude and longitude at a resolution much higher than the one of observations. We do so chiefly because we have no knowledge a priori of the number and timing of plate-motion changes that actually occurred over the period spanned by reconstructed finite rotations. In fact, we cast these as free parameters of each model within the ensemble [20] (trans-dimensional approach) and refer to them as change points, because the trends of residual angle, longitude and latitude change at these geological instants. This allows us to take into account also the uncertainty on the geomagnetic reversal timescale used to time finite rotations. Similarly, the uncertainty of each model is parameterized within the model itself [19] (hierarchical approach) to account for our ignorance on the noise magnitude, and thus on how close to the data a given model should be in order for the latter to be considered a faithful realization of the true temporal trends. As Euler vectors may change position or angular velocity independently, the sole constraint we impose on the ensemble consists of requiring latitude and longitude to change simultaneously, but independently from the residual angle. We then assign each model with a probability of representing the true temporal changes [17] (Bayesian approach), defined from the misfit between model and the data (Methods). That is, we estimate the chance of each model being the solution we seek, given the data we have. This is often referred to as posterior probability [26] . A trans-dimensional Monte Carlo Markov chain ( Methods ) allows us to efficiently sample the posterior probability density function (PDF) of the model ensemble in the vicinity of the true solution. At first glance, models with a greater number of change points may seem prone to fit the data better, hence yielding higher posterior probability with respect to simpler (that is, less change points) models. However, it is well established that trans-dimensional Bayesian inference follows the principle of 'natural parsimony' [18] , where preference always falls on the least complex explanation of observations. Reduction of finite-rotations noise We obtain the most likely realizations of the true residual angle, longitude and latitude as weighted averages of the PDFs (solid lines in Fig. 2a,b and Supplementary Figs S3a–b and S4a–b ). From the ensemble solution, we also construct posterior probabilities of change points in the temporal trends of residual angle and longitude/latitude at any time over the interval spanned by finite rotations. These are obtained by counting the recurrence of a change point within the entire ensemble. At times when most models consistently feature a change point, the probability that a true change occurred, given the data, is highest. On the contrary, when only few models feature a change point the posterior probability is low ( Fig. 2c and Supplementary Figs S3c and S4c ). Note that for all three spreading systems, probability maxima of the residual angle coincide with those of longitude/latitude, thus reinforcing our inference that the ensemble mean captures the reflection of true plate-motion changes in the finite-rotation series. More importantly, we find that any two consecutive, significant plate-motion changes are separate in time by intervals no shorter than ∼ 5 Myr ( Fig. 2c and Supplementary Figs S3c and S4c ). This finding reconciles observed lithosphere kinematics with inferences on the dynamics, as it is in good agreement with the typical timescale of the fastest geological processes generating torques upon plates, such as the descent of slabs into the Earth's mantle [15] , the interaction of mantle flow and plume heads with the lithosphere base [3] , [27] , [28] and the influence of surface processes on the tectonics of plate margins [29] among others. 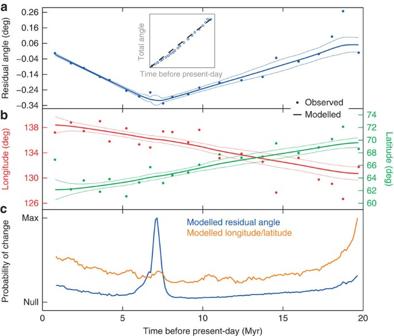Figure 2: Reconstructed and modelled Eurasian/North America finite rotations. (a) Residual angle (computed as departure from the linear trend imposed by the oldest reconstructed finite rotation—inset) observed (dots) and modelled (thick line) in a trans-dimensional hierarchical Bayesian framework. Modelled residual angle is computed as weighted average of the ensemble PDF. Thin lines limit the confidence region of the PDF average. (b) Longitude (in red) and latitude (in green) of finite-rotation poles observed (dots) and modelled (thick line) in a trans-dimensional hierarchical Bayesian framework. Thin lines limit the confidence regions of the PDF averages. (c) Probability of a change point in the temporal trend of modelled residual angle (in blue) and longitude/latitude (in orange). Note that the increased change probability for modelled longitude/latitude towards the present day and∼20 Ma is an artefact due to the truncation of the temporal series. Figure 2: Reconstructed and modelled Eurasian/North America finite rotations. ( a ) Residual angle (computed as departure from the linear trend imposed by the oldest reconstructed finite rotation—inset) observed (dots) and modelled (thick line) in a trans-dimensional hierarchical Bayesian framework. Modelled residual angle is computed as weighted average of the ensemble PDF. Thin lines limit the confidence region of the PDF average. ( b ) Longitude (in red) and latitude (in green) of finite-rotation poles observed (dots) and modelled (thick line) in a trans-dimensional hierarchical Bayesian framework. Thin lines limit the confidence regions of the PDF averages. ( c ) Probability of a change point in the temporal trend of modelled residual angle (in blue) and longitude/latitude (in orange). Note that the increased change probability for modelled longitude/latitude towards the present day and ∼ 20 Ma is an artefact due to the truncation of the temporal series. Full size image From the ensemble of modelled finite rotations, which carry no loss of temporal resolution compared to observations, we compute Euler vectors and their covariance matrices ( Supplementary Data 1 ) for the relative motion between spreading plates at the native temporal resolution of observations ( Fig. 3a and Supplementary Figs S5a and S6a ). We then map these into spreading rates across the associated ridges ( Fig. 3b and Supplementary Figs S5b and S6b ). A comparison with spreading rates from the original reconstructed finite rotations (black profile) reveals that the ensemble mean preserves the general trend of spreading evolution through time, but the kinematic changes requiring implausible torques upon plates over short geological periods are removed from temporal trends. A synthetic test where the true signal is known shows the efficiency of the Bayesian framework in retrieving plate kinematics compared with a more classical smoothing by average ( Methods ). Here we emphasize, however, that averaging always requires an arbitrary choice of the length of the averaging time-window, thus yielding different results depending on such length. 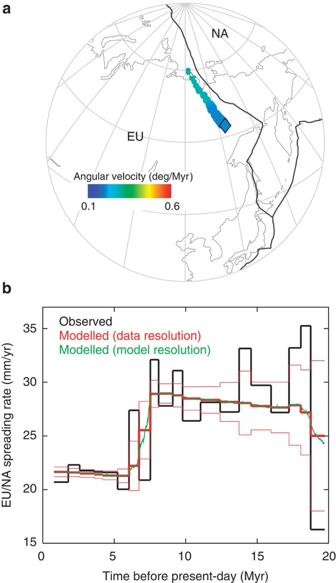Figure 3: Modelled plate kinematics. (a) Euler poles (dots) for the relative motion of the Eurasian plate (EU) with respect to fixed North America plate (NA) since∼20 Ma, reconstructed from modelled finite-rotations discretized according to the temporal resolution of observations. Euler poles are colour-coded according to their angular velocity. Note the same colour bar ofFig. 1a. Symbol size increases from the oldest to the youngest (shown as diamond) Euler pole. EU and NA plate margins are in black. Coastlines are in grey. (b) EU/NA spreading rates at (28°W, 45°N) from observed (in black) and modelled (in green) Euler vectors. In thick red are modelled spreading rates discretized at the temporal resolution of observations. Uncertainty ranges from the model ensemble are in thin red. Figure 3: Modelled plate kinematics. ( a ) Euler poles (dots) for the relative motion of the Eurasian plate (EU) with respect to fixed North America plate (NA) since ∼ 20 Ma, reconstructed from modelled finite-rotations discretized according to the temporal resolution of observations. Euler poles are colour-coded according to their angular velocity. Note the same colour bar of Fig. 1a . Symbol size increases from the oldest to the youngest (shown as diamond) Euler pole. EU and NA plate margins are in black. Coastlines are in grey. ( b ) EU/NA spreading rates at (28°W, 45°N) from observed (in black) and modelled (in green) Euler vectors. In thick red are modelled spreading rates discretized at the temporal resolution of observations. Uncertainty ranges from the model ensemble are in thin red. Full size image The peculiarity of plate motions to change on typical timescales no shorter than a few Myr has significant implication for the figure of present-day lithosphere kinematics derived from space geodesy, for which continuous measurements, mainly from the global positioning system [23] , [24] , are recorded since the advent of geodesy in the Earth Sciences about two decades ago [22] . To date, it remains unclear for how long in the geological past geodetically-derived plate motions remained stable, something that limits our ability to make inferences on the recent dynamics of the lithosphere. Our modelled Euler vectors sample with confidence the kinematics of the associated spreading systems over the past 20 to 40 Myr, and thus provide some insight. We analyse the frequency content of spreading-rate temporal series: First, we apply a low-pass period filter that removes any oscillatory contribution whose period is longer than a given cut-off value. Next, we compute the integral of the filtered spreading rates. We do so for progressively higher cut-off periods, therefore measuring how much is left of the original spreading-rate series after filtering (green profiles in Fig. 4 and Supplementary Figs S7 and S8 ). Naturally, if the original temporal series contains no or very little contributions at periods equal or shorter than the cut-off, the integral of its filtered image will be close zero. Instead, as the cut-off period progressively falls into the range of typical wavelengths of spreading-rate variations, we expect the integral of the filtered image to increase. Eventually, the integral will remain constant to its maximum value for cut-off periods longer than the longest period contributing to the spreading-rate series. 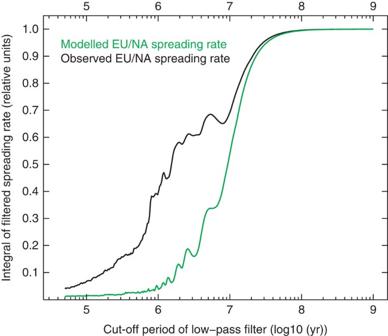Figure 4: Spectral analysis of spreading rates. In green, integral (relative units) of Eurasia/North America (EU/NA) spreading rates (green profile inFig. 3b), filtered at progressively higher cut-off periods. In black, the same analysis performed on noisy observed spreading rates (black profile inFig. 3b). Figure 4: Spectral analysis of spreading rates. In green, integral (relative units) of Eurasia/North America (EU/NA) spreading rates (green profile in Fig. 3b ), filtered at progressively higher cut-off periods. In black, the same analysis performed on noisy observed spreading rates (black profile in Fig. 3b ). Full size image We find that <5% of the spreading-rate temporal changes occurs at periods <1 Myr, and that the bulk of temporal changes feature periods longer than 30 to 50 Myr ( Fig. 4 and Supplementary Figs S7 and S8 ). From this analysis we conclude that true plate motions are likely not to have changed significantly over time intervals shorter than ∼ 1 Myr, indicating that the figure of geodetically established plate motions must have remained stable far longer than ever thought. Note that the presence of noise in the original finite rotations prevents this type of analysis, primarily because it enhances intrinsic first-order discontinuities (that is, jumps) in spreading rates and therefore introduces artificial low-period components, known as Gibbs phenomenon (black profiles in Fig. 4 and Supplementary Figs S7 and S8 ). Consequently, noise would lead one to erroneously conclude that plate motions change significantly (up to ∼ 50%) over periods shorter than ∼ 1 Myr. As we anticipate the body of high-temporal-resolution finite rotations to grow at fast pace in the years to come, our study provides the opportunity to efficiently reduce noise from these data sets, therefore isolating true plate motions and their temporal changes. Trans-dimensional hierarchical model parameterization We construct one ensemble for each of the finite-rotation observables (residual angle, longitude or latitude), for each of the spreading plate-pairs considered (EU/NA, IN/SO and PA/AN). Within any ensemble, each model features a number of points representing instants, over the time period spanned by finite rotations, where the trend of finite-rotation observables (residual angle, longitude or latitude) changes. We refer to these as change points. The values assumed by each model at its own change points are initially selected in a random manner. In between any two consecutive change points the model varies linearly. The number of change points of each model is itself a free parameter of the model, therefore it may vary from one another. These features are evident in Supplementary Fig. S9 , where we show a sample of the IN/SO residual-angle ensemble. The observed temporal trend is also shown for comparison. Each model of the ensemble also features its own uncertainty that is proportional, through a positively defined scaling factor, to the uncertainty associated with observations. The value of the scaling factor is also a free parameter of the model, and may vary from one another. Bayesian inference In Bayesian inference the solution sought is not a single best-fitting model. Rather it is the weighted mean of a large (order of millions) ensemble of models. Model weights are distributed according to the posterior PDF, which represent the probability that a model is a realisation of the true observable, given the measurements. To obtain the posterior PDF we use Bayes theorem [17] and combine prior information about the model—that is, information we have before having made any measurements—with the observed data: ,where a / b means a given, or conditional on, b - that is, the probability of having a when b is fixed. m is the vector of the model parameters (that is, number and position of change points plus uncertainty) and d is a vector defined by the observed data (that is, residual angle, longitude and latitude of finite-rotations data sets). The term p ( d / m ) is the likelihood, or probability, of observing the measured data given a theoretical model for the temporal trend of finite rotations. The likelihood is simply defined by a least square misfit function given by the distance between observations and synthetic data estimated from a given model: where g ( m ) i is the i -th data point estimated from a given model m , and σ i is the s.d. of an assumed random Gaussian noise for the i -th data point (note that we also assume noise to be uncorrelated between any two data points). The term p ( m ) is the prior probability density of m —that is, what we know about the model m before measuring the data d . Here, we assume unobtrusive prior knowledge by setting priors to uniform distribution with relatively wide bounds. The posterior PDF is then reconstructed by efficiently sampling the model space through the trans-dimensional generalisation of the well-known Metropolis–Hasting algorithm [30] , [31] named reversible jump Markov chain Monte Carlo sampler. Finally, we obtain modelled finite rotations from the means of residual angle, longitude and latitude ensembles. Efficiency of the trans-dimensional hierarchical Bayesian We test the efficiency of the trans-dimensional hierarchical Bayesian framework in retrieving true plate motions through a synthetic test. For simplicity, we assume that the rotation pole for the relative motion between two given plates is known without uncertainty and remains fixed. The angular velocity, instead, varies through time with a known pattern that we impose (black envelope in Supplementary Fig. S10a–d ). In our test such temporal series is deemed as true plate motion. Note that we explicitly cast two events of plate-motion change—that is, jumps in angular velocity—at 4 Myr as well as around 9 Myr before present day. We then add white Gaussian noise to the temporal series of true plate motion (grey envelope in Supplementary Fig. S10a–d ). From the pattern of noisy angular velocity we compute synthetic noisy finite rotations, which are meant to mimic the result of hypothetical magnetic surveys of the ocean-floor. The efficiency in reducing noise and identifying true plate motions is linked to how well the magnitude and timing of the temporal changes initially cast in the true plate motion are retrieved from noisy synthetic finite-rotations. We apply the Bayesian framework to the temporal series of noisy synthetic finite rotations, to obtain modelled finite rotations. From these, we then compute the modelled temporal series of plate motion (red envelope in Supplementary Fig. S10a ). Results show clearly that the Bayesian framework retrieves the timing and magnitude of true plate-motion changes quite effectively. We compare this result to the angular velocity obtained after averaging noisy synthetic measurements over intervals of 2 Myr (green in Supplementary Fig. S10b ), 3.5 Myr (green in Supplementary Fig. S10c ) and 5 Myr (green in Supplementary Fig. S10d ). It is evident from this comparison that one never retrieves either the timing or the magnitude—in some cases both—of true plate-motion changes through averaging as efficiently as through the Bayesian framework. More importantly, averaging does not yield a unique solution, as it depends strongly on the time interval over which plate motions are averaged. Therefore, there are chiefly two reasons why we prefer the Bayesian framework over smoothing to reduce noise from finite-rotation measurements: There is no systematic criterion to decide what type of smoothing one should apply—In particular, whether one should average noisy measurements over 2, 3 or more millions of years—and any reasonable choice would virtually lead to a different solution. On the contrary, the Bayesian framework requires no such choice to be made, therefore ensuring uniqueness of the solution. Averaging a temporal series of experimental measurements comes by definition at the cost of decreasing the resolution at which measurements are originally made. Instead, no loss of resolution compared with measurements is associated with the Bayesian framework. If one also considers that magnetic surveys of the ocean-floor are very expensive mainly because of ship-time, then our preference falls on the Bayesian framework, particularly because we know upfront that the solution obtained from smoothing is comparatively not as precise. How to cite this article: Iaffaldano, G. et al . Reconstructing plate-motion changes in the presence of finite-rotations noise. Nat. Commun. 3:1048 doi: 10.1038/ncomms2051 (2012).